Sustaining the Internet with hyperbolic mapping The Internet infrastructure is severely stressed. Rapidly growing overheads associated with the primary function of the Internet—routing information packets between any two computers in the world—cause concerns among Internet experts that the existing Internet routing architecture may not sustain even another decade. In this paper, we present a method to map the Internet to a hyperbolic space. Guided by a constructed map, which we release with this paper, Internet routing exhibits scaling properties that are theoretically close to the best possible, thus resolving serious scaling limitations that the Internet faces today. Besides this immediate practical viability, our network mapping method can provide a different perspective on the community structure in complex networks. In the information age, the Internet is becoming a de facto public good, akin to roads, airports or any other critical infrastructure [1] . According to the Internet World Stats, more than a thousand million people are estimated to use the Internet every day, to communicate, search for information, share data or do business. Online social networks are becoming an integral part of human social activities, increasingly affecting human psychology [2] . Underlying all these processes is the Internet infrastructure, composed, on a large scale, of connections between autonomous systems (ASs). An AS is, roughly, a part of the Internet owned and administered by the same organization [3] . ASs range in size from small companies, or even private users, to huge international corporations. No central Internet authority exists that dictates to any AS what other ASs to connect to. Connections between ASs are results of local independent decisions based on business agreements between AS pairs. This lack of centralized engineering control makes the Internet a truly self-organized system, and poses many scientific challenges. The one we address here is the sustainability of Internet growth. The Internet has been growing fast according to all measures [4] , [5] . For example, the number of ASs increases by ~2,400 every year [4] . Despite its growth, the Internet must sustainably perform its primary task—routing information packets between any two computers in the world. But can this function be really sustained? To route information to a given destination in the Internet today, all ASs must collectively discover the best path to each possible destination, based on the current state of the global Internet topology. As the number of destinations grows quickly, the amount of information each AS has to maintain becomes a serious scalability concern, endangering the performance and stability of the Internet [6] . Worse yet, the Internet is not static. Its topology changes constantly because of the failure of existing links and nodes, or because of the appearance of new ones. Each time such a change occurs anywhere in the Internet, the information about this event must be diffused to all ASs, which have to quickly process it to recompute new best routes. The constantly increasing size and dynamics of the Internet thus leads to immense and quickly growing routing overheads, causing concerns among Internet experts that the existing Internet routing architecture may not sustain even another decade [6] , [7] , [8] , [9] ; parts of the Internet have started sinking into black holes already [10] . The scaling limitations of the existing Internet routing stem from the requirement to have a current state of the Internet topology distributed globally. Such global knowledge is unavoidable, as routing has no source of information other than the network topology. Routing in these conditions is equivalent to routing using a hypothetical road atlas, which has no geographical information but merely lists road network links, which are pairs of connected road intersections, abstractly identified. This analogy with road routing suggests that there are better ways to find paths in networks. Let us assume that we want to travel from one geographical place to another. Given the geographical coordinates of our starting point and destination, we can readily determine which direction brings us closer to our destination. We see that a coordinate system in a geometric space, coupled with a representation of the world in this space, drastically simplifies our routing task. Thus, for simple and efficient network routing we need a map. Constructing such a map for the Internet boils down to assigning to each AS its coordinates in some geometric space, and then using this space to forward information packets in the right directions towards their destinations. Greedy forwarding implements this routing in the right direction: on reading the destination address in the packet, the current packet holder forwards the packet to its neighbour that is closest to the destination in the space. This greedy strategy to reach a destination is efficient only if the network map is congruent with the network topology. In the analogy with road routing, for example, this congruency condition means that there should exist a road path that stays approximately close to the geographical geodesic between the trip's starting and ending points. If the congruency condition holds, then the advantage of greedy forwarding is twofold. First, the only information that ASs must maintain is the coordinates of their neighbours. That is, ASs do not have to keep any perdestination information. Second, once ASs are given their coordinates, these coordinates do not change on topological changes of the Internet. Therefore, ASs do not have to exchange any information about ever-changing Internet topology. Taken together, these two improvements essentially eliminate the two scaling limitations mentioned above. In our recent work [11] , [12] , [13] , [14] , [15] , we have shown that greedy forwarding is indeed efficient in Internet-like synthetic networks embedded in geometric spaces, and that this efficiency is maximized if the space is hyperbolic. However, putting these ideas in practice needs a crucial piece of information: a map of the real Internet in a hyperbolic space. Here, we present a method to find such a map. Our method uses statistical inference techniques to find coordinates for each AS in the hyperbolic space underlying the Internet. Guided by the inferred coordinates, greedy forwarding in the Internet achieves efficiency and robustness, similar to those in synthetic networks. We also find that the method maps geo-politically close ASs close to each other in the hyperbolic space. This finding suggests that our mapping method can be used for soft community detection in real networks, where by soft communities we mean groups of geometrically close nodes. To build a geographical map, one first has to model the Earth surface, for example, by assuming that it is a sphere. Similarly, we also need a geometric model of the Internet space to build our map. The simplest candidate space is also a sphere, or even a circle, on which nodes are uniformly distributed and connected by an edge, with probability p ( d ) decreasing as a function of distance d between nodes, conceptually similar to random geometric graphs [16] . However, this model fails to capture basic properties of the Internet topology, including its scale-free node degree distribution. In an earlier study [17] , we showed that to generate realistic network topologies in this geometric approach, we first have to assign to nodes their expected degrees κ drawn from a power-law distribution, and then connect pairs of nodes with expected degrees κ and κ ′ with probability p ( χ ), where χ is distance d rescaled by the product of the expected degrees, χ~–d/ ( κκ′ ). We thus have a hybrid model that mixes geometry and topology—geometric characteristics, distances d used in random geometric graphs, come in tandem with topological characteristics, expected degrees κ used in classical configuration models of random power-law graphs [18] . If we associate the expected degree κ of a node with its mass, then the connection probability p ( d/ ( κκ′ )), which is a measure of the interaction strength between two nodes, resembles Newton's law of gravitation. Therefore, we call this model Newtonian. However, according to Einstein, we can treat gravity in purely geometric terms if we accept that the space is no longer flat, that is, if it is non-Euclidean. Following this philosophy we showed in an earlier study [13] that the Newtonian model is isomorphic to a purely geometric network model, with node degrees transformed into a geometric coordinate, making the space hyperbolic, that is, negatively curved. We call this model Einsteinian. 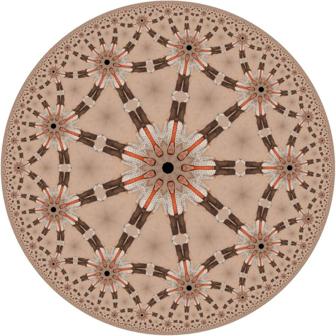Figure 1: Hyperbolic geometry at a glance. The exponentially growing number of people lying on the hyperbolic floor illustrates the exponential expansion of the hyperbolic space. All people are of the same hyperbolic size. The Poincaré tool developed by Bill Horn is used to construct the tessellation of the hyperbolic plane in the Poincaré disc model with the Schläfli symbol {9, 3}, rendering an image of the last author. The main property of hyperbolic geometry is the exponential expansion of space illustrated in Figure 1 . For example, the area A ( r ) of a two-dimensional hyperbolic disc of radius r grows with r as A ( r )~ e r . 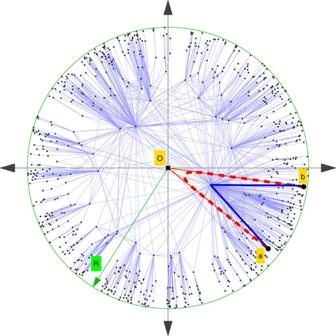Figure 2: Synthetic network in the Einsteinian model. The modelled network illustrates the connection between hyperbolic geometry and scale-free topology of complex networks. All nodes lie within a hyperbolic disc of radiusR. The radial node density grows exponentially with the distance from the originO, whereas the average degree of nodes exponentially decreases. This combination of the exponentially increasing node density and exponentially decreasing average degree yields a power-law degree distribution in the network. The red lines show triangleOabmade of the hyperbolic geodesics (that is, shortest paths in the hyperbolic space) connecting originOand two nodesaandb. Geodesicsandare the solid red lines, whereas geodesicis the dashed curve. The thick blue links show the shortest path between nodesaandbin the network. Consequently, the uniform node density in a hyperbolic space appears as exponentially growing with the distance r from the origin (see Figure 2, illustrating the Einsteinian model). In the model, nodes are indeed distributed (quasi-)uniformly on a hyperbolic disc, and one can show 13 that the resulting average degree of nodes exponentially decreases with r . This combination of two exponentials, node density and average degree, leads to the emergence of a scale-free degree distribution in the network. The model is described in the Methods section, and can generate synthetic scale-free networks with any power-law degree distribution exponent and any clustering. Given a real network, our network mapping method, also in the Methods section, reverts the network synthesis in the model. The method uses statistical inference techniques to identify the hyperbolic coordinates for each node in the given network, which would maximize the likelihood that the network is generated by the model. Specifically, the method attempts to find node positions such that the resulting empirical probability of node connections as a function of the hyperbolic distance between nodes would be congruent with the theoretical connection probability in the model. Figure 1: Hyperbolic geometry at a glance. The exponentially growing number of people lying on the hyperbolic floor illustrates the exponential expansion of the hyperbolic space. All people are of the same hyperbolic size. The Poincaré tool developed by Bill Horn is used to construct the tessellation of the hyperbolic plane in the Poincaré disc model with the Schläfli symbol {9, 3}, rendering an image of the last author. Full size image Figure 2: Synthetic network in the Einsteinian model. The modelled network illustrates the connection between hyperbolic geometry and scale-free topology of complex networks. All nodes lie within a hyperbolic disc of radius R . The radial node density grows exponentially with the distance from the origin O , whereas the average degree of nodes exponentially decreases. This combination of the exponentially increasing node density and exponentially decreasing average degree yields a power-law degree distribution in the network. The red lines show triangle Oab made of the hyperbolic geodesics (that is, shortest paths in the hyperbolic space) connecting origin O and two nodes a and b . Geodesics and are the solid red lines, whereas geodesic is the dashed curve. The thick blue links show the shortest path between nodes a and b in the network. 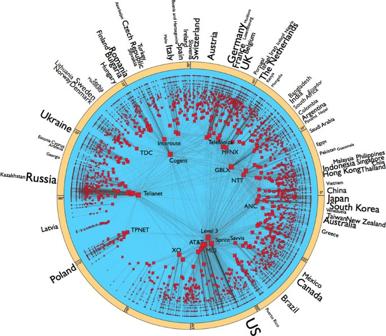Figure 3: Hyperbolic atlas of the Internet. The Internet's hyperbolic map is similar to a synthetic Einsteinian network inFigure 2. The size of AS nodes is proportional to the logarithm of their degrees. For the sake of clarity, only ASs with a degree above 3 and only the connections with probabilityp(x)>0.5 given by Equation (4) of the Methods section are shown. The font size of the country names is proportional to the logarithm of the number of ASs that the country has. Only the names of countries with more than 10 ASs are included. The methods used to map ASs to their countries are described inSupplementary Methods. Full size image Mapping results We apply our mapping method to the Internet AS topology extracted from the Archipelago project data [19] in June 2009, and visualize the results in Figure 3 . We observe striking similarity between this visualization and the synthetic Einsteinian network in Figure 2 . 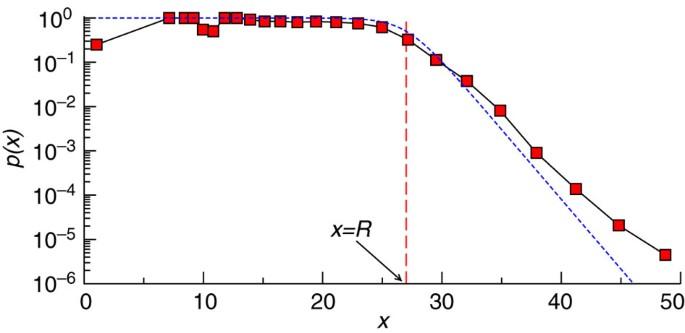Figure 4: Empirical versus theoretical connection probability. Hyperbolic mapping of the Internet is successful, as the empirical connection probability between ASs of degree larger than 2 in the map closely follows the Einsteinian model prediction. The whole range of hyperbolic distancesis binned, and for each bin the ratio of the number of connected AS pairs to the total number of AS pairs falling within this bin is shown. The distances between AS pairs are computed using Equation (3). The blue dashed line is the connection probability given by Equation (4) withR=27 andT=0.69, which are the values used by the mapping method. To confirm that the Internet map we have obtained is indeed congruent with the Einsteinian model, we juxtapose in Figure 4 the empirical connection probability between ASs in the obtained Internet map against the theoretical one in Equation (4) of the Methods section. We observe a clear similarity between the two. Neither is the sphere a perfect model of the Earth nor is the Einsteinian model an ideal abstraction of the Internet structure. Yet, the observed similarity between the empirical and theoretical connection probabilities in Figure 4 suggests that hyperbolic metric spaces are reasonable representations of the real Internet space. Figure 3: Hyperbolic atlas of the Internet. The Internet's hyperbolic map is similar to a synthetic Einsteinian network in Figure 2 . The size of AS nodes is proportional to the logarithm of their degrees. For the sake of clarity, only ASs with a degree above 3 and only the connections with probability p ( x )>0.5 given by Equation (4) of the Methods section are shown. The font size of the country names is proportional to the logarithm of the number of ASs that the country has. Only the names of countries with more than 10 ASs are included. The methods used to map ASs to their countries are described in Supplementary Methods . Full size image Figure 4: Empirical versus theoretical connection probability. Hyperbolic mapping of the Internet is successful, as the empirical connection probability between ASs of degree larger than 2 in the map closely follows the Einsteinian model prediction. The whole range of hyperbolic distances is binned, and for each bin the ratio of the number of connected AS pairs to the total number of AS pairs falling within this bin is shown. The distances between AS pairs are computed using Equation (3). The blue dashed line is the connection probability given by Equation (4) with R =27 and T =0.69, which are the values used by the mapping method. 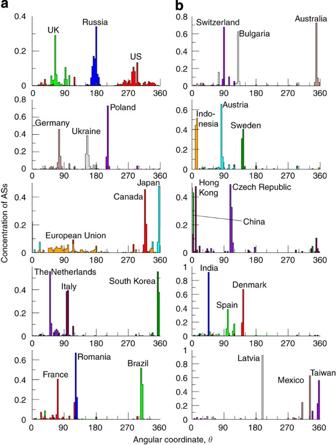Figure 5: Angular positions of ASs belonging to the same country. Hyperbolic mapping of the Internet yields meaningful results, as ASs belonging to the same country are mapped close to each other. The angular distributions of ASs in the 30 largest countries in the world are shown. The 'size' of the country is the number of ASs it has. Columnacorresponds to the first 15 countries and columnbto the next 15. The graph shows the percentage of ASs per bin of size 3.6°. For the majority of countries, their ASs are localized in narrow regions. Exceptions are the United States, the European Union and the United Kingdom. The first two exceptions are because of the significant geographic spread of ASs belonging to the United States or the European Union, the latter actually representing not one country but a collection of countries. Full size image To investigate further the connections between the obtained map and Internet reality, we show in Figure 3 the average angular position of all ASs belonging to the same country, whereas in Figure 5 we draw the angular distributions of those ASs. Surprisingly, we find that even though our mapping method is completely geography agnostic, it discovers meaningful groups or communities of ASs belonging to the same country. Furthermore, in Figure 3, we find many cases of geographically or politically close countries placed close to each other in our hyperbolic map. The explanation of these surprising effects is rooted in the peculiar nature of our mapping method. If ASs belonging to the same country, geographic region or geo-political or economic group are connected more densely to each other than to the rest of the world, then this higher connection density translates to a higher attractive force that tries to place all such ASs close to each other in our map. Indeed, the term p ( x i j ) a i j in Equation (7) of the Methods section corresponds to the attractive force between connected nodes, whereas the term [ 1 - p ( x i j ) ] 1 - a i j is the repulsive force between disconnected ones. This peculiar interplay between attraction within densely connected regions and repulsion across sparsely connected zones effectively maps the ASs belonging to densely connected AS groups closely. These observations build our confidence that our mapping method provides meaningful results reflecting peculiarities of the real Internet structure, and suggest that the method can be adapted to discover the community structure [20] , [21] , [22] in other complex networks. Figure 5: Angular positions of ASs belonging to the same country. Hyperbolic mapping of the Internet yields meaningful results, as ASs belonging to the same country are mapped close to each other. The angular distributions of ASs in the 30 largest countries in the world are shown. The 'size' of the country is the number of ASs it has. Column a corresponds to the first 15 countries and column b to the next 15. The graph shows the percentage of ASs per bin of size 3.6°. For the majority of countries, their ASs are localized in narrow regions. Exceptions are the United States, the European Union and the United Kingdom. The first two exceptions are because of the significant geographic spread of ASs belonging to the United States or the European Union, the latter actually representing not one country but a collection of countries. Full size image Routing results The obtained Internet map is ready for greedy forwarding. An AS holding a packet reads its destination AS coordinates, computes the hyperbolic distances between this destination and each of its AS neighbours using Equation (3) of the Methods section and forwards the packet to the neighbour closest to the destination. To evaluate the performance of this process, we perform greedy forwarding from each source to each destination AS, and compute several performance metrics. The first metric is success ratio, which is the percentage of greedy paths that successfully reach their destinations. Not all paths are expected to be successful, as some might run into local minima. For example, an AS might forward a packet to its neighbour who sends the packet back to the same AS, in which case the packet will never reach the destination. We declare a path unsuccessful if the packet is sent to the same AS twice. The average success ratio of simple greedy forwarding in our Internet map is remarkably high, 97%, and more sophisticated greedy forwarding techniques, such as those described in Cvetkovski and Crovella study [23] , can boost it to 100%. Given the discussed connections between our Internet map and geography, one may conjecture that greedy forwarding simply mimics geographical routing following the geographically shortest paths. However, this conjecture is not true. Geography is reflected in our map only along the angular coordinate, whereas the radial coordinate is a function of the AS degree, making the space hyperbolic (see the Methods section). The geographical space is not hyperbolic, and if we use it for greedy forwarding, we obtain a much lower success ratio of approximately 14%. We also tested modified geographic routing that tries to intelligently use AS degrees, in the spirit of our Einsteinian model. Nevertheless, this modification, although improving the success ratio to 30%, still falls short compared with the results obtained using our hyperbolic map. The details of these experiments with geographical routing can be found in Supplementary Methods . The second metric is stretch, which tells us how much longer the greedy paths are compared with the shortest paths in the Internet topology. The average stretch is low, 1.1. The average hop-wise length of the shortest paths between selected sources and destinations is 3.49, so that the average length of greedy paths is 3.86. The low value of stretch indicates that greedy paths are close to optimal, that is, they are the shortest paths. The shortest path between nodes a and b in Figure 2 , for example, is also the path found by greedy forwarding. Somewhat unexpectedly, the greedy stretch is asymptotically optimal, that is, equal to 1, in scale-free, strongly clustered networks, regardless of what underlying space is used for greedy forwarding [12] . Low stretch also implies that greedy forwarding causes approximately the same traffic load on nodes as shortest-path forwarding. Given that shortest-path forwarding does not lead to high traffic load in scale-free networks [24] , this finding allays concerns that hyperbolic forwarding may cause traffic congestion abnormalities [25] (see Supplementary Methods ). The two metrics above characterize the performance of greedy forwarding in the static Internet topology. More important than that is how greedy forwarding performs in the dynamic topology, in which links and nodes can fail. 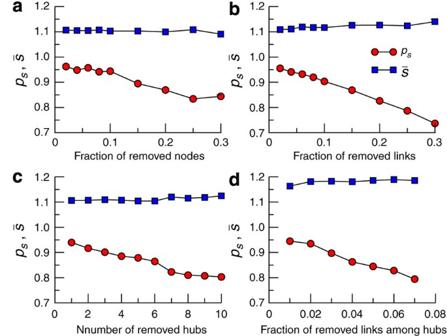Figure 6: Greedy forwarding in the mapped Internet. Greedy forwarding performs almost optimally in the mapped Internet, as indicated by the success ratio,ps, and average stretch,, after removal of a given fraction of AS nodes (panela) or links (panelb). Bottom plots show these two metrics after removing a number of the highest-degree nodes (panelc), and a fraction of links among highest-degree nodes (paneld). The links are first ranked by the product of node degrees that they connect, and then a fraction of top-ranked links are removed. The giant connected component is still present after all removals, but it drops to 85% of the original graph after the removal of 10 hubs. We randomly select a percentage of links and nodes, remove them from the mapped Internet, recompute the success ratio and stretch after the removal and finally present the result in the top plots of Figure 6 . Even on simultaneous failures of up to 10% of AS links or nodes—catastrophic events never happened in Internet history—we observe only minor de-gradation of the performance of greedy forwarding. That is, even catastrophic levels of damage to the Internet do not significantly affect the performance of greedy forwarding, even though no AS changes its position on the hyperbolic map. A widely popularized feature of complex networks is their robustness with respect to random failures, and the lethality of failures of highest-degree hubs [26] , [27] . As expected, we observe in the bottom plots of Figure 6 that removals of such hubs have a more detrimental effect on greedy forwarding as well. However, targeted removal of highest-degree ASs in the Internet is a rather unrealistic scenario, as these large ASs consist of thousands of routers the simultaneous failure of which is a very rare and unlikely event. The explanation for the surprising efficiency of greedy forwarding with respect to random failures lies in the unique combination of the following two properties exhibited by scale-free, strongly clustered networks: high path diversity [24] , and congruency between hyperbolic geodesics and topologically shortest paths [13] , [15] . The latter is illustrated by the similar path patterns of the hyperbolic geodesic and topologically shortest path between nodes a and b in Figure 2 : they both first go to the high-degree core of the network, and then exit it in the appropriate direction to the destination. Owing to high path diversity, there are many disjoint shortest paths between the same source and destination, and thanks to the congruency, they all stay close to the corresponding hyperbolic geodesics. Link and node failures affect some shortest paths, but others remain, and greedy forwarding can still find them using the same hyperbolic map. Figure 6: Greedy forwarding in the mapped Internet. Greedy forwarding performs almost optimally in the mapped Internet, as indicated by the success ratio, p s , and average stretch, , after removal of a given fraction of AS nodes (panel a ) or links (panel b ). Bottom plots show these two metrics after removing a number of the highest-degree nodes (panel c ), and a fraction of links among highest-degree nodes (panel d ). The links are first ranked by the product of node degrees that they connect, and then a fraction of top-ranked links are removed. The giant connected component is still present after all removals, but it drops to 85% of the original graph after the removal of 10 hubs. Full size image Another form of Internet dynamics is its rapid growth over years [4] , [5] , [28] , [29] . We map the Internet of January 2007 to its hyperbolic space using the same mapping method, and then replay the historical growth of the Internet up to June 2009 with an interval of 3 months. During this two and a half year replay, we keep the AS coordinates, as soon as they are computed, fixed once and forever, whereas the ASs joining the Internet anew, after June 2007, compute their coordinates using a variation of the mapping method that requires only local topological information (see Supplementary Methods ). 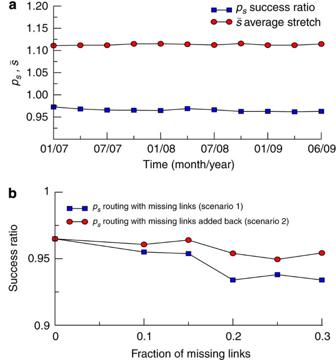Figure 7: Performance of greedy forwarding during the replayed historical growth of the Internet (a), and success ratio as a function of the fraction of missing links (b). The initial map quality degrades very slowly with time (a). The Internet is fully mapped only once, in June 2007. The ASs that appear after that date compute their coordinates using only local topological information. Once the coordinates of an AS are computed, they are fixed forever. The average success ratiopsand stretchfor greedy forwarding in the resulting collection of maps are shown for each snapshot at 3-month intervals, starting from January 2007 and ending in June 2009. SeeSupplementary Methodsfor further details. The success ratio also degrades slowly with the number of missing links (b), and if these missed links are added back, the success ratio increases—the larger the number of missing links, the more the success ratio increases. Scenario 1 (blue squares): (i) a fraction of random links among nodes of degree above 5 in the Internet are removed (30% of removed links in this subgraph correspond to 14% of the total number of links in the Internet); (ii) the resulting graph with emulated missing links is hyperbolically mapped using the same mapping method; (iii) the success ratio in the resulting map is computed. Scenario 2 (red circles): (i) and (ii) are the same as in Scenario 1; (iii) the removed links are added back; (iv) the success ratio is computed. SeeSupplementary Methodsfor further details. In Figure 7a, we show the performance of greedy forwarding in the resulting maps at each time step, and observe only minor performance degradation, even over long time scales. In a nutshell, the existing AS coordinates are essentially static, as once computed they can stay the same for years. Figure 7: Performance of greedy forwarding during the replayed historical growth of the Internet ( a ), and success ratio as a function of the fraction of missing links ( b ). The initial map quality degrades very slowly with time ( a ). The Internet is fully mapped only once, in June 2007. The ASs that appear after that date compute their coordinates using only local topological information. Once the coordinates of an AS are computed, they are fixed forever. The average success ratio p s and stretch for greedy forwarding in the resulting collection of maps are shown for each snapshot at 3-month intervals, starting from January 2007 and ending in June 2009. See Supplementary Methods for further details. The success ratio also degrades slowly with the number of missing links ( b ), and if these missed links are added back, the success ratio increases—the larger the number of missing links, the more the success ratio increases. Scenario 1 (blue squares): (i) a fraction of random links among nodes of degree above 5 in the Internet are removed (30% of removed links in this subgraph correspond to 14% of the total number of links in the Internet); (ii) the resulting graph with emulated missing links is hyperbolically mapped using the same mapping method; (iii) the success ratio in the resulting map is computed. Scenario 2 (red circles): (i) and (ii) are the same as in Scenario 1; (iii) the removed links are added back; (iv) the success ratio is computed. See Supplementary Methods for further details. Full size image Existing Internet topology measurements including the Archipelago data [19] are known to be incomplete and miss some AS links [28] , [29] . Therefore, a natural question is how this missing information affects the quality of the constructed map, and the performance of greedy forwarding in it. Intuitively, as the performance of greedy forwarding is robust with respect to link removals, we might expect it to be robust with respect to missing links as well. Moreover, if the constructed map is used in practice, then greedy forwarding will see and use those links that topology measurements do not see. We might thus also intuitively expect greedy forwarding to perform better in practice than we report in this section, simply because those missing links, when used by greedy forwarding, would provide additional shortcuts between potentially remote ASs. We confirm this intuition in Figure 7b with experiments emulating the missing link issue. The success ratio degrades only slowly as a function of the fraction of missing links, whereas if we add the emulated missing links back, then the success ratio increases as expected. Therefore, the routing results reported here should actually be considered as lower bounds for greedy routing performance that can be achieved in practice using the constructed hyperbolic Internet map. We have constructed a hyperbolic map of the Internet, and release this map as part of the Supplementary Data set . The map can be used for essentially infinitely scalable Internet routing. The amount of routing information that ASs must maintain is proportional to the AS degree, which is theoretically best possible as ASs must always keep some information about their neighbours. Routing communication overheads are also minimized, as ASs do not exchange any routing information on dynamic changes of the AS topology. The presented solution thus achieves routing efficiency that is theoretically close to optimal, and resolves serious scaling limitations that the Internet faces today. The mapping method we have used is generic, and can be applied to other complex networks with underlying metric structures and heterogeneous degree distributions. We showed in an earlier study [17] that a good indicator for the presence of an underlying metric structure is self-similarity of clustering in the network, whereas in an earlier study [13] we showed that as soon as a metric space is present, and the network has a heterogeneous degree distribution, the metric distances can be rescaled such that the underlying geometry is effectively hyperbolic. Roughly, self-similar clustering is responsible for the metric structure along the angular coordinate, whereas degree heterogeneity adds the radial dimension and makes the space hyperbolic. Applied to other networks, our mapping method can provide a different perspective on the community structure in networks. Instead of trying to split nodes into discrete community sets [20] , [21] , [22] , it would naturally yield a continuous measure of similarity between nodes on the basis of hyperbolic distances. More similar nodes would be located closer to each other, and form zones of higher connectivity density. Thereafter, it would be up to an experimenter to define communities, if needed, as histograms of the node density in the hyperbolic space. The spectrum of potential applications of this network-mapping geometrization agenda is wide. Network mapping can reveal geometric forces effectively driving information signalling in the network; examples include the brain [30] and cell signalling networks [31] . One can then potentially predict what network perturbations drive these networks to failure, such as brain disorders or cancer. Other applications range from recommender systems [32] , in which the right measure of similarity between consumers is a key, to epidemic spreading [33] and information theory of networks [34] . We have shown that the Internet hyperbolic map is remarkably robust with respect to even substantial perturbations of the Internet topology, implying that this map is essentially static. It does not significantly depend on topology dynamics, and can thus be computed only once. This property is desirable in view of long running times intrinsic to likelihood maximization algorithms. Our method improves their running times drastically, and the Internet map computations take approximately a day on a modern computer. However, for substantially larger networks, the running times may still be prohibitive even for one-time mapping. Therefore, alternative methods for network mapping, not relying on likelihood maximization, are highly desirable, and our work in this direction is underway. The Einsteinian and Newtonian models of complex networks To synthesize a network with our Einsteinian model, one has to first specify any desired network size N , as well as average degree , average clustering and exponent γ >2 of the power-law distribution P ( k ) of node degrees k , P ( k )~ k − γ . Equipped with these target properties of the network topology, we first distribute N nodes (quasi-)uniformly within a hyperbolic disc of radius R =2log( N / c ), where c is given by and is a function of . In the hyperbolic plane, the quasi-uniform node density means that the node angular coordinates are distributed uniformly, whereas their radial coordinates are distributed with density where α =( γ −1)/2. Once all nodes are in place, specified by their assigned coordinates, the hyperbolic distance x ij between each pair of nodes i and j located at ( r i , θ i ) and ( r j , θ j ) is computed using the hyperbolic law of cosines where Δ θ ij is the angle between segments connecting the origin and points i and j . On distributing nodes over the disc as described, we form scale-free networks in the model by connecting each pair of nodes i and j located at hyperbolic distance x ij with the connection probability almost identical to the Fermi-Dirac distribution in statistical mechanics. It depends only on hyperbolic distances x ij (link energies), the hyperbolic disc radius R (chemical potential) and parameter T ≥0 (temperature) controlling network clustering. After each node pair is examined and connected with probability p ( x ij ), the network is formed and we can compute the average degree k ( r ) of nodes located at distance r from the origin. The result is which, combined with Equation (2), yields the target degree distribution P ( k ). The Newtonian model is isomorphic to the Einsteinian one through a simple change of variables reminiscent of Equation (5): where κ is the expected degree of a node in the Newtonian model, and κ 0 is the minimum expected degree. See Krioukov et al . [13] for further details. The mapping method As our goal is to build a realistic Internet map, ready for routing and other applications, we have to find for each AS its radial and angular coordinates ( r , θ ), maximizing the efficiency of greedy forwarding. This specific task of maximizing greedy forwarding efficiency calls for a mapping method different from existing techniques on embedding Internet distances and graphs [35] , [36] , [37] . In view of our previous findings [11] , [12] , [13] , [14] , [15] that greedy forwarding is exceptionally efficient in Internet-resembling synthetic networks, and that this efficiency is maximized in the Einsteinian model, our strategy for the Internet map construction is to maximize the congruency between the map and the model. In statistical inference [38] , this goal is equivalent to maximizing the likelihood that the observed data, that is, the Internet topology, has been produced by the model. This likelihood is given by where the elements a ij of the Internet adjacency matrix are equal to 1 whenever there exists a connection between ASs i and j , and to 0 otherwise. Whereas the adjacency matrix represents the observed data, the connection probability p ( x ij ) depends, by means of Equations (4, 3), on the AS coordinates ( r , θ ), which we try to infer. Our best estimate for these coordinates is then those maximizing the likelihood in Equation (7). Although there are plenty of methods to find maximum-likelihood solutions, for example, the Metropolis–Hastings algorithm [39] , they perform poorly and do not scale well on large data sets with abundant local maxima, which is the case with the Internet. Therefore, as important as a likelihood maximization method is a heuristic approach helping the maximization algorithm to find the optimal solution in a reasonable amount of time and with reasonable computational resources. Our method is based on the following remarkable property of networks in our model; the same property holds for the Internet [17] . Let G be a given network with average degree and power-law degree distribution P ( k )~ k − γ , and let G ( k T ) be G 's subgraph composed of nodes with degree larger than some threshold k T , along with the connections among these nodes. The average degree in G ( k T ) is then given by . [17] In scale-free networks with exponent γ between 2 and 3, this internal average degree is thus a growing function of k T , which implies that subgraphs made of high-degree nodes almost surely form a single connected component. Using this property, along with the statistical independence of the graph edges, it becomes possible to infer coordinates of ASs in G ( k T ) ignoring the remainder of the AS graph. This property is practically important because the size of G ( k T ) decreases very fast as k T increases, which speeds up likelihood maximization algorithms tremendously. In a nutshell, our method starts with a subgraph G ( k T ) small enough for standard maximization algorithms being able to reliably and quickly infer the coordinates of ASs in G ( k T ). Once these are found, we gradually increase k T to iteratively add layers of lower-degree ASs. While doing so, we use the already inferred AS coordinates as a reference frame to assign initial coordinates to newly added ASs. This initial coordinate assignment significantly improves the convergence time of maximization algorithms. All other details of our mapping method can be found in Supplementary Methods . The archipelago Internet topology We use the AS Internet topology of June 2009 extracted from data collected by the archipelago active measurement infrastructure developed by Cooperative Association for Internet Data Analysis [19] . The AS topology contains 23752 ASs and 58416 AS links, yielding the average AS degree = 4.92 . The maximum AS degree is k max =2778. The average clustering measured over ASs of degree larger than 1 is = 0.61, yielding temperature T =0.69, and hyperbolic disc radius R =27. The exponent of the power-law AS degree distribution is γ =2.1. This Internet topology is available as part of the Supplementary Data set , along with the hyperbolic Internet map. How to cite this article: Boguñá, M. et al . Sustaining the Internet with hyperbolic mapping. Nat. Commun. 1:62 doi: 10.1038/ncomms1063 (2010).